Ultrasensitive magnetic field detection using a single artificial atom Efficient detection of magnetic fields is central to many areas of research and technology. High-sensitivity detectors are commonly built using direct-current superconducting quantum interference devices or atomic systems. Here we use a single artificial atom to implement an ultrasensitive magnetometer with micron range size. The artificial atom, a superconducting two-level system, is operated similarly to atom and diamond nitrogen-vacancy centre-based magnetometers. The high sensitivity results from quantum coherence combined with strong coupling to magnetic field. We obtain a sensitivity of 3.3 pT Hz −1/2 for a frequency at 10 MHz. We discuss feasible improvements to increase sensitivity by one order of magnitude. The intrinsic sensitivity of this detector at frequencies in the 100 kHz–10 MHz range compares favourably with direct-current superconducting quantum interference devices and atomic magnetometers of equivalent spatial resolution. This result illustrates the potential of artificial quantum systems for sensitive detection and related applications. Sensitive physical measurements are an essential component of modern science and technology. In particular, detection of magnetic fields is an area of wide interest, with various applications including medical imaging, geomagnetics, non-destructive materials evaluation, scanning probe microscopy, and electrical measurements [1] , [2] . Magnetic field sensors are also enabling tools for fundamental studies of magnetism [3] , spin dynamics [4] , fundamental symmetries [2] and mechanical motion [5] , [6] . Sensitive tools to detect magnetic fields are diverse and include direct-current superconducting quantum interference devices (DC-SQUIDs) [1] , atomic magnetometers [2] , Hall probes [7] and magnetostrictive sensors [8] . DC-SQUIDs have been established for a long time as very sensitive magnetometers [1] . In recent years, significant advances in atomic control led to the development of atomic magnetometers, which presently compete with DC-SQUIDs for magnetic field detection and have the convenience of operation in a room temperature environment [2] . Atomic magnetometers rely on the measurement of the effect of the field on the coherent dynamics of an ensemble of atoms. A detection method similar to atomic magnetometry can be implemented using nitrogen-vacancy defects (NV centres) in diamond crystals [9] . Magnetometers based on single NV centres [10] , [11] have been demonstrated and shown to have interesting prospects as high-spatial-resolution high-sensitivity detectors. The principle of our approach follows closely that of magnetometry based on vapour cells or NV centres [2] , [9] . The method employs a Ramsey interferometry sequence. The first step is initialization of the spin in a superposition of the up and down states with respect to a reference axis. Precession due to an applied magnetic field for a duration τ around time t leads to an accumulated phase , with μ the magnetic moment and B ( t ) the time-dependent component of the magnetic field along the reference axis. Next, the spin is rotated with a coherent control pulse, so that the projection along the reference axis depends on φ ( t , τ ), hence on the magnetic field. A single measurement produces a result r =±1, corresponding to the two spin states. For N repetitions of the sequence, the average value of the measurement 〈 r 〉=sin φ and the standard deviation is . The minimum detectable magnetic field difference, corresponding to a signal to noise ratio of 1, is . This can be expressed as , with T rep the repetition time of the procedure described above and T = NT rep the total measurement time. The sensitivity can thus be expressed as the quantity δB min , which has units of T Hz −1/2 . The sensitivity increases with the time τ as long as the evolution is fully coherent; with decoherence taken into account, the optimum is reached when τ is of the order of the Ramsey coherence time T 2 * . In existing magnetometers based on this principle, the two spin states of interest are hyperfine or Zeeman levels in alkali atoms [2] or spin sublevels of the ground state in NV centres in diamond [9] . Detection is done most commonly using an ensemble of atoms/defects. With N at atoms, sensitivity is further enhanced by a factor = the volume and n the density of the cloud. The dependence of sensitivity implies that there is a tradeoff between sensitivity and spatial resolution. The same tradeoff also appears in magnetic field sensors based on DC-SQUIDs [1] . In this paper, we demonstrate ultra-high sensitivity detection of alternating current (AC) magnetic fields using a single artificial atom. The artificial atom is a persistent current qubit (PCQ)—a micron-sized superconducting ring with Josephson junctions [12] . This system has been studied extensively for quantum computing applications [13] . Owing to the interaction with its solid state environment, the PCQ has a coherence time that is shorter than in typical atomic systems. The lower coherence time is unfavourable for sensitive detection. However, this drawback is compensated for by the large coupling to magnetic field, typically five orders of magnitude larger than in atomic systems. To optimize magnetic field detection sensitivity, we use an operation mode based on detection of correlation of qubit measurement results. We find a sensitivity of 3.3 pT Hz −1/2 for operation at 10 MHz. The detection bandwidth around a centre frequency of 8 MHz reaches 1 MHz, limited at present by the overhead time introduced by measurement. The measured sensitivity is comparable with state of the art magnetometers based on DC-SQDUIDs or atoms/NV centres of equivalent spatial resolution. We present a theoretical analysis which shows that one order of magnitude further improvement is possible with feasible changes in the detection scheme. Our results demonstrate the potential of artificial quantum systems for high-sensitivity low-backaction detection. Coherent control and measurement of the qubit state The artificial atom used in our experiments for magnetic field detection, a PCQ, is a superconducting loop with three Josephson junctions, shown in Fig. 1 . The qubit is operated in a dilution refrigerator at a temperature of 43 mK. The qubit Hamiltonian is given by , where Φ is the magnetic flux applied to the qubit ring, Φ 0 = h /2 e is the flux quantum, and h Δ is the minimum energy-level splitting of the qubit, which occurs at the symmetry point Φ=Φ 0 /2 (see Fig. 1d ). This representation of the Hamiltonian uses two states with persistent current ± I p flowing in the qubit ring. The effective magnetic moment of the qubit is with hν ge the energy-level difference between the excited (e) and ground (g) states and B =Φ/ A qb the magnetic field applied to the qubit ring; A qb is the qubit loop area. The magnetic moment is given by . For our qubit, characterized by I p =140 nA, A qb =24.5 μm 2 and Δ=9.82 GHz, and operated at ν ge =11.39GHz, μ reaches the value 3.8 × 10 5 μ B . This large magnetic moment enables a large sensitivity, despite the coherence time of the PCQ being shorter than in typical atomic systems [2] , [9] . We note that a different method to use a PCQ for magnetometry, based on susceptibility of a qubit as opposed to quantum coherent dynamics, was discussed in [14] ; the predicted sensitivity is lower than for the detection scheme we discuss here. 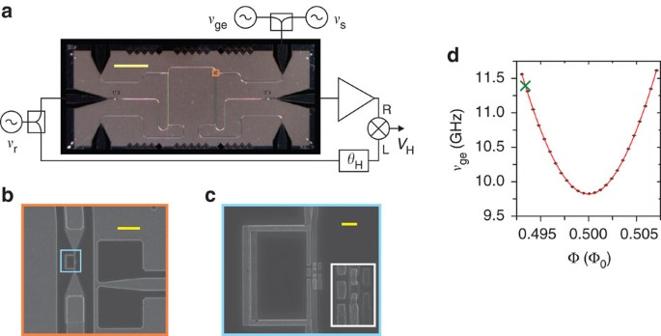Figure 1: Qubit control/readout circuit and spectroscopy. (a) Optical microscope image of a microfabricated device nominally identical to the device used in this work and schematic representation of the control and readout circuit. Scale bar, 1 mm. The qubit is at the position indicated by the orange rectangle. A coplanar waveguide resonator is used for qubit readout: microwaves at frequencyνrare applied at the input port (left) and the transmitted wave at the output port (right) is amplified and down converted to determine the homodyne voltageVH. The detected quadrature can be adjusted by changing the phaseθHof the local oscillator. A coplanar waveguide (top right port) is used to send microwave signals close to the frequencyνgeof the qubit transition, to implement coherent control, as well as to apply the AC voltage at frequencyνsto induce the magnetic field to be detected. (b) Zoom of the region indicated by the orange rectangle in (a). Scale bar, 10 μm. The qubit is the rectangular loop, coupled to the centre line of the resonator. On the right, the termination of the line for qubit control and AC field generation (connected to top right port in a) is shown. (c) Zoom of the region indicated by the blue rectangle in b. Scale bar, 1 μm. The bottom right inset shows details of the Josephson junctions. (d) Qubit spectroscopy measurement. The continuous line is a fit with the expression, which allows extracting the qubit parameters Δ andIpgiven in the text. The cross indicates the position, atνge=11.39 GHz, where the AC magnetic field measurements are performed. Figure 1: Qubit control/readout circuit and spectroscopy. ( a ) Optical microscope image of a microfabricated device nominally identical to the device used in this work and schematic representation of the control and readout circuit. Scale bar, 1 mm. The qubit is at the position indicated by the orange rectangle. A coplanar waveguide resonator is used for qubit readout: microwaves at frequency ν r are applied at the input port (left) and the transmitted wave at the output port (right) is amplified and down converted to determine the homodyne voltage V H . The detected quadrature can be adjusted by changing the phase θ H of the local oscillator. A coplanar waveguide (top right port) is used to send microwave signals close to the frequency ν ge of the qubit transition, to implement coherent control, as well as to apply the AC voltage at frequency ν s to induce the magnetic field to be detected. ( b ) Zoom of the region indicated by the orange rectangle in ( a ). Scale bar, 10 μm. The qubit is the rectangular loop, coupled to the centre line of the resonator. On the right, the termination of the line for qubit control and AC field generation (connected to top right port in a) is shown. ( c ) Zoom of the region indicated by the blue rectangle in b. Scale bar, 1 μm. The bottom right inset shows details of the Josephson junctions. ( d ) Qubit spectroscopy measurement. The continuous line is a fit with the expression , which allows extracting the qubit parameters Δ and I p given in the text. The cross indicates the position, at ν ge =11.39 GHz, where the AC magnetic field measurements are performed. Full size image Control of the state of the PCQ is done by an applied magnetic flux Φ. We bias the qubit with a flux Φ( t )=Φ b + δ Φ( t ), where Φ b is a static bias flux produced by an external coil and δ Φ( t ) is a fast varying flux coupled to the qubit via a coplanar waveguide terminated by an inductance (see Fig. 1a ). We can write the qubit Hamiltonian as , where τ x and τ z are Pauli operators in the energy eigenbasis and ɛ b =arctan( I p (Φ b −Φ 0 /2)/( h Δ)). Coherent qubit control is implemented by applying a flux δ Φ( t )= δ Φ 0 ( t )cos(2 πν ge t − β ( t )) with the amplitude δ Φ 0 ( t ) and the phase β ( t ) slow (compared with ) functions of time. In the frame rotating at the qubit frequency, the Hamiltonian is given by . Here is the Pauli operator along an axis in the xy plane at an angle β ( t ) with the x axis. Below, we use to denote a rotation of angle θ around an axis defined by the vector . Quantum measurement of the PCQ state is performed by using a circuit-quantum electrodynamics set-up in the dispersive regime [15] , [16] , [17] , [18] . The qubit is inductively coupled to a superconducting resonator, with a resonance frequency ν res =6.602 GHz, and quality factor Q =4,000 defined by coupling to the input and output ports. The resonance frequency of the cavity is modified due to the presence of the qubit by an amount that depends on the state of the qubit. Consequently, the complex transmission coefficient at frequencies close to the resonance frequency ν res is strongly qubit state dependent. To measure the state of the qubit, a microwave readout pulse of duration T r and frequency ν r = ν res is sent to the resonator. The complex amplitude of the transmitted pulse, as determined in a homodyne measurement [19] , is averaged over the duration T r of the readout pulse. In Fig. 2 we present the results of the qubit measurement. We only show one quadrature of the transmitted voltage, V H ; the axis for this quadrature is chosen such that it optimizes the measured signal (see Fig. 1a ). The qubit is prepared either in the ground state, by allowing for a waiting time much longer than the energy relaxation time T 1 =1.3 μs ( Fig. 2a ) or in the excited state by including a π x pulse before readout ( Fig. 2b ). The distribution of the values of the homodyne voltage V H is plotted in Fig. 2c and d , respectively. The distribution is bimodal, with the two modes corresponding to the qubit energy eigenstates. A threshold is used to separate the distribution into a part labelled r =−1 and the complementary part labelled r =1. The threshold is chosen so that it optimizes the readout contrast, which is the difference of the conditional probabilities P ( r =−1|e)− P ( r =−1|g). The maximum contrast is 66%. This high readout fidelity is essential for the sensitivity of the detector. 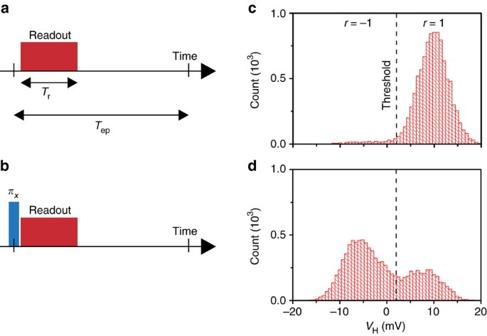Figure 2: Characterization of readout efficiency for the persistent current qubit. (a,b) Protocol used for characterization of readout for the ground state (a) and the excited state (b). The excited state is prepared by applying aπpulse prior to qubit readout. The readout time isTr=300 ns. The repetition timeTrep=10 μs is chosen significantly longer than the qubit relaxation timeT1. (c,d) Histograms of the homodyne voltage valuesVHfor preparation in the ground state (c) and the excited state (d), for 104repetitions. The vertical dashed line indicates the position of the threshold used to separate values labelledr=1 andr=−1, which are associated with the ground and excited states of the qubit, respectively. Figure 2: Characterization of readout efficiency for the persistent current qubit. ( a , b ) Protocol used for characterization of readout for the ground state ( a ) and the excited state ( b ). The excited state is prepared by applying a π pulse prior to qubit readout. The readout time is T r =300 ns. The repetition time T rep =10 μs is chosen significantly longer than the qubit relaxation time T 1 . ( c , d ) Histograms of the homodyne voltage values V H for preparation in the ground state ( c ) and the excited state ( d ), for 10 4 repetitions. The vertical dashed line indicates the position of the threshold used to separate values labelled r =1 and r =−1, which are associated with the ground and excited states of the qubit, respectively. Full size image Procedure for AC magnetic field detection In typical magnetometers, as introduced above, free precession in a magnetic field is employed. This procedure is adapted to detection of low-frequency fields, with frequency ranging from DC to 1/2 T rep , where T rep is the repetition time of the control/measurement procedure. For a PCQ operated in this way, the detection sensitivity is low due to the short Ramsey coherence time T 2 * , which is limited by low-frequency magnetic flux noise [20] , [21] . Low-frequency noise sets the ultimate limit for measurement of low-frequency fields, a situation also encountered for DC-SQUIDs [1] . For this reason, we focus here on detection of AC magnetic fields. The procedure is illustrated in Fig. 3a . The qubit is controlled using a series of spin-echo pulse sequences, with each sequence consisting of pulses applied at times t − τ /2, t and t + τ /2, respectively. The qubit phase precession for the sequence at time t is given by (see Supplementary Fig. S1 ). The amplitude B ac of an AC field B(t)= B ac cos(2 πν s t + α ) can be detected optimally when and α =0. In general, applying pulses with fixed τ is sufficient to detect the two quadratures of a field at frequency τ −1 with a band ranging from DC up to b max /2. The bandwidth b max is smaller than τ −1 and further limited by 1/ T rep when sampling issues are taken into account (see Supplementary Fig. S2 and Supplementary Methods ). Therefore, the useful detection frequency band is ( τ −1 − b max /2, τ −1 + b max /2). The advantage of detection using spin-echo pulses as opposed to free precession is that the corresponding coherence time, T 2 , is significantly longer than the Ramsey time T 2 * (ref. 20 ), which renders the sensitivity to AC field higher than for low-frequency fields. 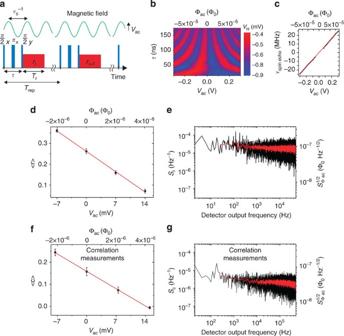Figure 3: Characterization of detection sensitivity. (a) Qubit control and measurement sequence. A spin-echo sequence of durationτis applied with a repetition timeTrep. A magnetic field with amplitude proportional to the control voltageVacis applied at frequencyνsin phase with the spin-echo pulses. In each experiment, a numberNsof series, each withNmmeasurements, is used to extract the average detector output and the noise spectral density (see theMethodssection for details). (b) Qubit evolution versus the amplitudeVacand the spin-echo timeτ. (c) The frequency of the oscillations in b versus amplitudeVac, for the range |Vac|>60 mV, where the frequency determination is reliable. The continuous line is a linear fit yielding the ∂vspin–echo/∂Vac=81.6 kHz mV−1factor used for data calibration. (d,e) Experiments withTrep=10 μs andτ=100 ns. For each value ofVac, the detector outputris analysed forNs=4 series, each withNm=50,000 measurements. (d) The average and the standard deviation (error bars) of theNsseries averages. The continuous line is a linear fit. (e) The noise spectral density (black) forVac=0 mV and an adjacent points average over a 50-Hz window (red). (f,g) Experiments withTrep=1 μs andτ=100 ns. For each value ofVac, the correlatorci=riri−1is analysed forNs=4 series ofNm=50,000 measurements. (f) The average and the s.d. (error bars) of theNsseries averages. The continuous line is a linear fit. (g) The spectral density of the noise of the detector output (black) forVac=0 mV and an adjacent points average over a 500-Hz window (red). Figure 3: Characterization of detection sensitivity. ( a ) Qubit control and measurement sequence. A spin-echo sequence of duration τ is applied with a repetition time T rep . A magnetic field with amplitude proportional to the control voltage V ac is applied at frequency ν s in phase with the spin-echo pulses. In each experiment, a number N s of series, each with N m measurements, is used to extract the average detector output and the noise spectral density (see the Methods section for details). ( b ) Qubit evolution versus the amplitude V ac and the spin-echo time τ . ( c ) The frequency of the oscillations in b versus amplitude V ac , for the range | V ac |>60 mV, where the frequency determination is reliable. The continuous line is a linear fit yielding the ∂ v spin–echo /∂ V ac =81.6 kHz mV −1 factor used for data calibration. ( d , e ) Experiments with T rep =10 μs and τ =100 ns. For each value of V ac , the detector output r is analysed for N s =4 series, each with N m =50,000 measurements. ( d ) The average and the standard deviation (error bars) of the N s series averages. The continuous line is a linear fit. ( e ) The noise spectral density (black) for V ac =0 mV and an adjacent points average over a 50-Hz window (red). ( f , g ) Experiments with T rep =1 μs and τ =100 ns. For each value of V ac , the correlator c i = r i r i −1 is analysed for N s =4 series of N m =50,000 measurements. ( f ) The average and the s.d. (error bars) of the N s series averages. The continuous line is a linear fit. ( g ) The spectral density of the noise of the detector output (black) for V ac =0 mV and an adjacent points average over a 500-Hz window (red). Full size image We focus first on experiments on detection at fixed frequency ν s = τ −1 , using the procedure shown in Fig. 3a . The magnetic field is induced by applying an AC voltage of amplitude V ac to the transmission line used for qubit control (see Fig. 1a ) and acts via the term δ Φ( t ) in the qubit Hamiltonian H qb ( t ). The resulting magnetic flux and field amplitudes are denoted by Φ ac and B ac , respectively. The phase accumulated during the spin-echo sequence is (see Supplementary Methods ). An oscillation in the qubit population versus time τ is expected, with a frequency . We indeed observe oscillations (see Fig. 3b ) with a frequency proportional to V ac (see Fig. 3c ). Field detection using qubit reset by energy relaxation We next proceed to the characterization of magnetic field sensitivity. The output of the detector is the noisy binary signal r . The noise in r reflects the stochastic nature of quantum measurement. In the following, we express the results of detection in terms of the magnetic flux Φ applied to the qubit, as this facilitates the comparison with DC-SQUIDs. The noise in r can be represented as an equivalent noise in the amplitude Φ ac of flux oscillations. The latter is characterized by the spectral density . Here S r is the single-sided spectral density of the noise in the qubit readout and is the transfer function of the detector, with 〈 r 〉 the average value of r . The transfer function can be expressed as . The factor is determined from the linear fit in Fig. 3d and is the ratio of the factor determined from qubit spectroscopy and of the factor determined from the data in Fig. 3c . In this way we determine the equivalent detector input noise fully from a set of measurable quantities, without any assumption on coupling of the field to the qubit. We note that 〈 r 〉≠0 at V ac =0, due to the measurement asymmetry (see histograms in Fig. 2c ). We use a spin-echo control sequence time τ =100 ns chosen to correspond approximately to the optimal value for the measured qubit coherence time T 2 * . We determined T 2 =126±7 ns by fitting the temporal decay of the spin-echo oscillation envelope with the function , with T 1 independently determined [20] . Figure 3e shows S r and for one value of V ac . We note that the noise depends very weakly on V ac as long as 〈r〉<<1, which is the case for all the detector operation conditions reported here. A theoretical calculation of the sensitivity taking into account the finite measurement fidelity and qubit decoherence predicts a flat noise spectrum with a value of (7.3±0.6) × 10 −8 Φ 0 Hz −1/2 , in good agreement with the experimentally measured value of 8.9 × 10 −8 Φ 0 Hz −1/2 at high frequency. In the low-frequency region, excess noise is observed due to electronics drifts and interference. For fast detection, the equivalent flux noise is largely dominated by the value in the high frequency limit. For magnetic field detection, the sensitivity can be expressed as , yielding . Field detection based on the correlation method The detection sensitivity obtained above is limited primarily by the large ratio T rep / τ , which is in turn due to imposing T rep >> T 1 in order to prepare the qubit by energy relaxation. To improve the detection efficiency, we use another method. We take as detector output not the series r i , but rather the series c i +1 = r i +1 r i . The usefulness of this method can be understood by considering the ideal case of projective measurements and very long relaxation time. If r i =1, c i +1 = r i +1 . If r i =−1, the qubit is prepared in the excited state; the probabilities to obtain results r i +1 =1 and r i +1 =−1 are reversed; this is compensated for automatically as c i +1 =− r i +1 . The correlator c i has the same statistical properties as r i in the previous method, which was based on qubit preparation by energy relaxation (see Supplementary Methods ). The advantage is that the repetition time is significantly reduced. With qubit energy relaxation during measurement [22] , [23] and finite projection fidelity, the effectiveness of this scheme is reduced, however, the lower repetition time makes the overall result significantly better. The repetition time of the sequence T rep is experimentally optimized to balance two competing effects: a long T rep results in additional qubit relaxation, which reduces qubit projection when r =−1; a short T rep leads to additional decoherence of the qubit, presumably due to photon number fluctuations in the resonator [24] . We analyse the data using a method fully analogous to the method discussed above, which employs qubit relaxation. The relevant data is shown in Fig. 3f . Similarly to the experiment presented in Fig. 3d , 〈 c 〉≠0 at V ac =0 is observed in Fig. 3f due to the measurement bias. A significant improvement of sensitivity is achieved compared with the result obtained using qubit reset by relaxation. The equivalent flux noise, taken as the average in the frequency range 1–100 kHz, is 3.9 × 10 −8 Φ 0 Hz −1/2 . We note that a minor reduction in the noise power is observed at frequencies above 100 kHz, which was confirmed by numerical simulations to be related to the asymmetry of the measurement as induced by energy relaxation [23] . Excess noise is observed at low frequency, however, the magnitude is significantly lower than that for the data shown in Fig. 3e , due to the fact that low-frequency fluctuations in the detection system are removed by using the correlations. The magnetic field detection sensitivity reaches . Detector frequency and amplitude response We next present experiments on wideband detection using the correlation method (see Fig. 4 ). We applied magnetic fields at different frequencies ν s , with a starting phase which is arbitrary at the beginning of each sequence. We extracted the noise power using the method explained above. For frequencies ν s in the band ( τ −1 −(2 T rep ) −1 , τ −1 +(2 T rep ) −1 ), a peak is observed at frequency | ν s − τ −1 | (see Fig. 4a ). For ν s outside this interval, a signal is detected for ν s in a bandwidth τ −1 around centre frequency τ −1 , however, undersampling will make this peak appear at a frequency translated to the detection band (see Supplementary Methods ); this is the case for ν s =8.990 MHz in Fig. 4a . We also characterized the amplitude response of the detector, at a frequency ν s =8.05 MHz, which is offset with respect the central frequency τ −1 ( Fig. 4b ). The response is linear, with a slope compatible with the conversion factor determined based on spin-echo measurements for ν s = τ −1 (see Supplementary Fig. S3 ). Finally, we performed an experiment in which we applied two tones at different frequencies, with the result shown in Fig. 4c . Additional experiments, characterizing the response to a change in the signal phase, are presented in Supplementary Fig. S4 . The combination of experiments presented in this section, demonstrating amplitude, frequency and phase response, indicates that realistic signals can be measured using our detector. 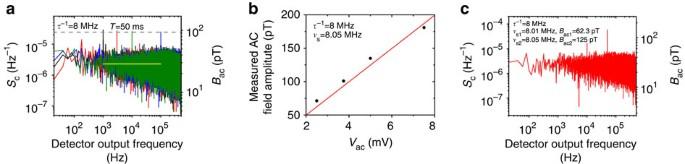Figure 4: Detection bandwidth around centre frequency. Detection of magnetic fields using the correlation method. The measurement sequence, shown inFigure 3a, has spin-echo timeτ=125 ns and repetition timeTrep=8τ=1 μs. We average the power spectral densityScoverNs=4 series, with each series lastingT=50 ms. (a) The power spectral densitySc(left vertical axis) and the corresponding AC amplitude (right vertical axis) is given for four measurements in which we applied a AC magnetic field of amplitudeBac=94 pT (Φac=1.08 × 10−6Φ0), indicated by the dashed grey line, and different frequenciesνs(black, red, blue and green traces are for 8.001, 8.003, 8.100 and 8.990 MHz, respectively). The continuous yellow line shows the average noise in the frequency band 1–100 kHz. (b) The amplitude of the measured AC field amplitude atνs=8.05 MHz is plotted as a function of the applied AC voltage amplitudeVac. The continuous line is the expected dependence, calculated based on the conversion factor that had been characterized independently. (c) The power spectral densitySc(left vertical axis) and the corresponding AC amplitude (right vertical axis) is shown for the case when a two-tone signal is applied to the detector, with frequencies and amplitudes as indicated in the legend. Figure 4: Detection bandwidth around centre frequency. Detection of magnetic fields using the correlation method. The measurement sequence, shown in Figure 3a , has spin-echo time τ =125 ns and repetition time T rep =8 τ =1 μs. We average the power spectral density S c over N s =4 series, with each series lasting T =50 ms. ( a ) The power spectral density S c (left vertical axis) and the corresponding AC amplitude (right vertical axis) is given for four measurements in which we applied a AC magnetic field of amplitude B ac =94 pT (Φ ac =1.08 × 10 −6 Φ 0 ), indicated by the dashed grey line, and different frequencies ν s (black, red, blue and green traces are for 8.001, 8.003, 8.100 and 8.990 MHz, respectively). The continuous yellow line shows the average noise in the frequency band 1–100 kHz. ( b ) The amplitude of the measured AC field amplitude at ν s =8.05 MHz is plotted as a function of the applied AC voltage amplitude V ac . The continuous line is the expected dependence, calculated based on the conversion factor that had been characterized independently. ( c ) The power spectral density S c (left vertical axis) and the corresponding AC amplitude (right vertical axis) is shown for the case when a two-tone signal is applied to the detector, with frequencies and amplitudes as indicated in the legend. Full size image These results establish the PCQ as an ultrasensitive AC magnetic field detector. In the following, a discussion is given on how our detector compares with other types of sensors. We focus on the comparison with DC-SQUIDs and atom-based detectors. For DC-SQUIDs, the most relevant figures of merit are the flux noise S Φ and the uncoupled energy sensitivity = S Φ /2 L , with L the loop inductance. The latter is particularly relevant for magnetometry [1] . For the PCQ in this experiment, and using L =27 pH we calculate . The SQUID in ref. 25 , operated at 290 mK, had . The SQUID in ref. 25 , operated at 25 mK, had . In both of these cases the energy sensitivity is the value measured at frequencies beyond kHz, where flux noise is negligible. The PCQ figures of merit in this experiment, which are still far from the theoretical limits that we discuss below, compare well with the optimized DC-SQUIDs in refs 25 and 26 . We also note that optimization of the uncoupled energy sensitivity of the PCQ can be done by increasing the loop inductance, as flux noise was observed in general not to scale up with loop size [20] ; this aspect is favourable for magnetometry [1] . The attained energy resolution and the prospects for further improvement, discussed below, raise interesting questions concerning the measurement backaction, as discussed for DC-SQUIDs in (refs 27 and 28 ). For a comparison with atomic and NV centre-based detectors, the most suitable figure of merit is the quantity δB min , which combines the sensitivity δB min and the detector volume V (ref. 2 ). Atomic magnetometers based on vapour cells have very high sensitivity, achieved usually with volumes of the order of 1 cm 3 , when sensitivities of the order of 0.1−1 fT Hz −1/2 (refs 3 and 29 ) are reached. When extrapolated to volumes of ≈1 μm 3 , corresponding to the PCQ detector used in this work, the ultimate theoretical limit to sensitivity is of the order of 1 pT Hz −1/2 (ref. 30 ). More recently, magnetic field detection based on cold atoms has been explored as well [31] , [32] . Using a Bose–Einstein condensate, a sensitivity of 8.3 pT Hz −1/2 was experimentally demonstrated in [31] for a measurement area of 120 μm 2 . The fundamental theoretical limit for sensing using a Bose–Einstein condensate with a resolution of a few micrometres [33] is in the pT Hz −1/2 range. We note that atomic magnetometers operate typically at low frequency, below 1 kHz; methods exist to extend the operation frequency to hundreds of kHz (ref. 34 ). NV centres in diamond [9] have recently emerged as an ultrasensitive method for magnetometry. They combine the possibility to work at room temperature and a spatial resolution that can be changed from the nanometre range (for single NV centre operation) [10] , [11] , [35] up to large scale by using a spin ensemble. Decoherence due to paramagnetic impurities limits the flux detection efficiency to 0.250 fT Hz −1/2 cm 3/2 , optimal for AC fields at frequencies of the order of 100 kHz (ref. 9 ), which results in a sensitivity of 100 pT Hz −1/2 for a detection volume of the order of 1 μm 3 . We discuss next the optimization of the detector sensitivity based on a set of realistic assumptions on parameters and feasible improvements of control and decoherence. At a given frequency ν s , optimizing the detection sensitivity requires tuning of the magnetic moment of the qubit. This can be achieved in situ by changing the qubit transition frequency ν ge . The dependence of the optimal sensitivity on frequency is calculated with the following assumptions. First, the persistent current I p and minimum energy-level splitting Δ are taken to have values as the PCQ in this experiment. Second, ideal projective measurements are used; projective measurements nearly reaching perfect fidelity have been demonstrated for superconducting qubits (see e.g., ref. 22 ). Third, the duty cycle ( τ / T rep ) is set equal to one. This can be achieved by shortening readout times, as enabled by nearly quantum-limited amplifiers [36] , [37] , and by replacing the spin-echo sequence with more complex control pulse schemes [9] , [21] , [35] . Last, qubit pure dephasing is assumed to be limited by 1/f flux noise (see ref. 20 ), with a spectral density given by (3.4 μΦ 0 ) 2 / f [Hz], which is the value that would explain the observed spin-echo decay time at ν ge =11.39 GHz in our experiment, if flux noise was the only noise contribution. This level of flux noise is larger than measured values in smaller area superconducting rings [20] , [21] , [38] . It is very likely that in our experiment the flux noise is significantly lower than this upper bound and that charge noise has a major role, due to the low Josephson energy in this device. Straightforward changes in design will allow reducing the influence of charge noise to negligible levels. With these assumptions taken into account, the calculated optimal sensitivity (see Supplementary Fig. S5 and Supplementary Methods ) is plotted in Fig. 5 for a PCQ with an energy relaxation time of 10 μs (attained in ref. 21 ) and for the case where relaxation is neglected. This calculation shows that with respect to the experimental results reported here, more than one order of magnitude of improvement is possible by feasible changes of the experimental set-up. The detection efficiency decreases with decreasing frequency, due to the ultimate limit imposed by 1/f noise. Nevertheless, this detector has a very high intrinsic sensitivity for measurements in the range from tens of kHz to tens of MHz. Possible future developments on increase of coherence times of superconducting qubits will increase the efficiency and the useful frequency range even further. 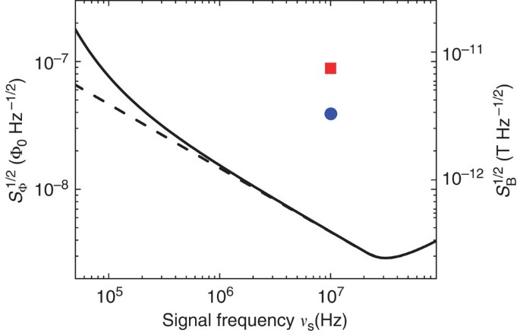Figure 5: Magnetic flux and field detection sensitivity for present results and ideal case. The calculated sensitivity for a PCQ for the case of ideal measurements and with a flux noise of 3.4 μΦ0Hz−1/2is given for the case of a relaxation timeT1=10 μs (continuous line) and for the case of negligible relaxation time (dashed line). The experimental results reported here are indicated by the red square (qubit reset done by energy relaxation) and blue dot (correlation measurements). Figure 5: Magnetic flux and field detection sensitivity for present results and ideal case. The calculated sensitivity for a PCQ for the case of ideal measurements and with a flux noise of 3.4 μΦ 0 Hz −1/2 is given for the case of a relaxation time T 1 =10 μs (continuous line) and for the case of negligible relaxation time (dashed line). The experimental results reported here are indicated by the red square (qubit reset done by energy relaxation) and blue dot (correlation measurements). Full size image In conclusion, we demonstrated a high-sensitivity magnetometer based on an artificial atom. The high magnetic field sensitivity combined with the micron spatial resolution is relevant to applications such as detection of electron spin resonance, scanning probe microscopy, and sensitive current and voltage amplifiers [1] . This detector is particularly interesting for exploring the dynamics of quantum systems at low temperatures with minimal backaction. The results here illustrate the potential that artificial quantum systems have for quantum sensing. Device fabrication The PCQ presented in this work is realized using a two-step fabrication process. In the first step, a resist layer is deposited on a silicon wafer and patterned using optical lithography to define all the device elements except the qubit. The resist is developed, then 200 nm of aluminium is evaporated onto the chip. Lifting off the resist removes Al from unpatterned regions. The second layer, which contains the qubit and the connexions to the central line of the coplanar waveguide resonator, is realized using standard shadow evaporation of aluminium. The Josephson junctions are formed by two aluminium layers, with thicknesses 40 and 65 nm, respectively, separated by an in situ grown thin aluminium oxide layer. Measurement set-up The experiments are performed in a dilution refrigerator, at a temperature of 43 mK (see [39] for additional details). The device is placed inside a copper box, connected to a printed circuit board by wire bonding. Connexions to transmission lines are done using microwave launchers on the printed circuit board. Magnetic shielding is implemented using three layers of high magnetic permeability material. The sample is connected to room temperature electronics using coaxial cables, which include various filter, isolation and amplification sections. The signal at the output port of the resonator is amplified using a low-noise high-electron-mobility transistor amplifier with a noise temperature of 4 K. Readout and control pulses are implemented using modulation of continuous-wave signals produced by synthesizers. Modulation signals are produced using arbitrary waveform generators with a time resolution of 1 ns (4 ns) for control (readout) pulses. The signal at the output of the resonator, amplified using the high-electron-mobility transistor amplifier, is further amplified using an amplification chain at room temperature, demodulated and digitized. The average of each readout output pulse is recorded for each repetition. The time series of the digital measurement output are used to extract average quantities and the noise power spectral density (PSD). Magnetic field biasing of the qubit is performed using a centimetre size coil attached to the copper box and fed by a current produced by a high-stability current source. Calculation of detector output noise from experiments The detector output noise, that is S r and S c for the two methods discussed in the text, respectively, is determined as follows. For a given detector pulse configuration and one given value of the V ac amplitude, N s series of measurement results, with each series formed of N m measurements, are acquired. The measurement results are denoted as r jk , with 1≤ j ≤ N s and 1≤ k ≤ N m . For each series we calculate the average r̄ j . The average and standard deviation of the set , plotted in Fig. 3d versus V ac , are used to extract the transfer function (∂〈 r 〉)/(∂V ac ). The spectral density of the r noise is calculated as , with T = N m T rep the total series time. We defined the discrete Fourier transform of the series R j as , for 1≤ k ≤ N m /2. The array S r ( k ) gives the single-sided spectral density of the noise, corresponding to frequencies f k = k /( N m T rep ). The S c noise is determined in an analogous manner. Relation between detector total noise and quadrature noise We consider a signal applied to the detector input of the form with f the magnetic flux Φ normalized to the flux quantum Φ 0 . In Supplementary Methods , section ‘Two-quadrature detection’, we discuss two protocols which allow for the measurement of the two quadratues, I and Q , of the signal. Using suitable transfer functions, as expressed by Supplementary equations S14 and S15 in Supplementary Methods , one can calculate , with I ( t ) and Q ( t ) the signal parts and I n ( t ) and Q n ( t ) the noisy parts. The noise component represents noise due to measurement randomness and possibly other components. We take in the following to be functions of time, although in the calculation of noise power spectra and Fourier components based on experiments, we use the discrete series of single measurement results. The two stochastic processes, I n ( t ) and Q n ( t ), are stationary: the correlation functions , with 〈〉 representing a process ensemble average, only depend on the time t ′. Stationarity is valid assuming that the measured fields are weak. Under the same assumption, the cross-correlation functions also depend only on the time difference t ′. The measured parameter calculated based on the measured quadratures can be written as . Here f ( t ) is the the signal defined in equation 1. The second part, is a random process. It is however not a stationary process, but a cyclostationary process [40] . The correlation function is periodic with t , with a period in given by 2 π / ω s 0 . In general, for two processes A ( t ) and B ( t ) for which the correlation function only depends on the time difference t ′, we define the cross-PSD as: When B is identical with A , this definition yields the regular PSD. For the process f n ( t ), which is not stationary, we consider the time averaged PSD. This is the relevant quantity when the noise is averaged over times long enough compared with the period 2 π / ω s 0 (ref. 41 ). The relation between the time averaged PSD S f , f , and the PSD and cross-PSD for the processes I n ( t ) and Q n ( t ) is given by: where we omitted the subscript n for quantities I n and Q n . All the cross-correlation spectral density functions vanish, as the two-quadrature measurement protocols discussed in the Supplementary Information Methods involve independent measurements. We next introduce the single-sided PSD for a random process A ( t ), defined for positive frequencies ω, as: For a frequency ω = ω s 0 + δ detuned from ω s 0 by an amount δ with | δ |< ω s 0 , and assuming that the spectrum of the quadrature noise is contained in the band (− ω s 0 , ω s 0 ), we obtain On the basis of equation 7, we can determine the relation between the equivalent input and the quadrature noise measured in our experiment. For a measurement in which only one quadrature, for definitiveness assumed to be I , is measured with repetition time T rep , let us denote the noise by . Consider next that the protocol is replaced by interleaved sampling ( Supplementary Information Methods , section ‘Two-quadrature detection’). Now each quadrature is measured with a repetition time 2 T rep . We have because the same total noise is spread over a smaller bandwidth, 1/2 T rep , as opposed to 1/ T rep . We also assume that the Q quadrature is measured in the same way, hence the output noise is the same. Using equation 7 we derive The consequence of relation 9 for the interpretation of the data in our experiment is very important. It tells us that the equivalent total detector noise input is properly described by the quantity , which is the quantity that we discuss in the paper. How to cite this article: Bal, M. et al . Ultrasensitive magnetic field detection using a single artificial atom. Nat. Commun. 3:1324 doi: 10.1038/ncomms2332 (2012).